Targeting matriptase in breast cancer abrogates tumour progression via impairment of stromal-epithelial growth factor signalling Matriptase is an epithelia-specific membrane-anchored serine protease that has received considerable attention in recent years because of its consistent dysregulation in human epithelial tumours, including breast cancer. Mice with reduced levels of matriptase display a significant delay in oncogene-induced mammary tumour formation and blunted tumour growth. The abated tumour growth is associated with a decrease in cancer cell proliferation. Here we demonstrate by genetic deletion and silencing that the proliferation impairment in matriptase-deficient breast cancer cells is caused by their inability to initiate activation of the c-Met signalling pathway in response to fibroblast-secreted pro-HGF. Similarly, inhibition of matriptase catalytic activity using a selective small-molecule inhibitor abrogates the activation of c-Met, Gab1 and AKT, in response to pro-HGF, which functionally leads to attenuated proliferation in breast carcinoma cells. We conclude that matriptase is critically involved in breast cancer progression and represents a potential therapeutic target in breast cancer. Pericellular proteases in cancer progression were previously considered to be primarily extracellular matrix protein-degrading enzymes. Although it is clear that proteases are involved in degradation events related to breaching the basement membrane and reorganization of the extracellular matrix during invasive growth, a more complex view of pericellular proteolysis has emerged in recent years. One concept in protease mechanistic research is that proteolytic modifications of targets, including activation of growth factors, are critically involved in carcinogenesis through activation of oncogenic signalling pathways. Importantly, tumour progression is characterized by a complex interplay between invading tumour cells and stromal cells, which includes paracrine interactions where growth factors secreted by stromal cells activate signalling pathways in the cancer cells. The type II transmembrane serine protease, matriptase, has been implicated in breast cancer since it was first discovered in breast cancer cell lines, and is highly expressed by the malignant cells in human breast carcinomas [1] , [2] , [3] , [4] , [5] . However, it is currently not known whether matriptase plays a critical role in breast cancer progression. One factor that has slowed advances on this front has been the perinatal lethality of matriptase-null mice, which has, thus far, precluded direct studies of matriptase loss-of-function in the mammary gland [6] , [7] . We circumvented this obstacle by employing a matriptase hypomorphic model with low levels of matriptase in the mammary gland. When crossed into the mouse mammary tumour virus (MMTV) Polyomavirus middle T (PymT) antigen genetic mammary tumour model, matriptase hypomorphic mice displayed a significant delay in tumour onset, as well as a decreased tumour burden and tumour multiplicity. The impaired growth was caused by a profound impairment of tumour cell proliferation. Hepatocyte growth factor or scatter factor (HGF or SF) is a pleiotropic , paracrine growth factor and key mediator of cell migration, proliferation, survival, motility and morphogenesis in epithelial cells [8] , [9] , [10] . HGF is biosynthesized as a single-chain zymogen-like inactive precursor (pro-HGF) and is proteolytically processed into its two-chain mature active form. The epithelial cell receptor, c-Met, binds pro-HGF or active HGF; however, only the active form elicits the c-Met signalling pathway [11] , [12] . Pro-HGF is secreted by mesenchymal cells, including fibroblasts and macrophages, in the breast. Importantly, c-Met is, like matriptase, expressed on the surface of mammary epithelial cells and breast carcinoma cells [5] , [13] . The HGF/c-Met signalling pathway is dysregulated in many cancer types, including breast cancer, and has been causally linked to breast carcinogenesis [13] , [14] , [15] , [16] , [17] . Thus, transgenic expression of HGF in mouse mammary glands causes formation of multifocal invasive tumours characterized by high-proliferation rates, and transgenic expression of activated c-Met leads to the development of mammary hyperplasia and malignant tumours [16] , [17] . Conversely, RNA interference (RNAi) or antibody mediated inhibition of c-Met in a variety of cancer cell lines, including breast, colon and multiple myeloma impairs cell proliferation and invasion, and increases chemosensitivity and radiosensitivity [18] , [19] , [20] , [21] . Since a key post-translational regulatory mechanism of oncogenic HGF/c-Met signalling is the proteolytic activation of pro-HGF, the identification of the critical activator(s) as potential targets for therapeutic intervention in cancer is important [22] . Here we demonstrate that matriptase is critically involved in mammary carcinogenesis and that the molecular mechanism through which matriptase exerts its pro-carcinogenic effects is by activation of pro-HGF on the cancer cell surface, leading to initiation of the c-Met signalling pathway and elicitation of mitogenic and invasive responses in breast cancer. Epithelial matriptase is upregulated in mammary carcinomas Transgenic MMTV-PymT mice are predisposed to develop multifocal mammary carcinomas with tumour progression that is very similar to that seen in human breast carcinomas [23] , [24] . To ensure that the mouse mammary cancer model closely mimics the observations in human breast cancer, matriptase expression in normal mammary glands and mammary tumours was characterized ( Fig. 1 ). A knock-in mouse with a promoterless β-galactosidase gene inserted into the endogenous matriptase gene was used as a unique tool for precise assessment of endogenous matriptase expression in the mammary gland by X-gal staining [25] , [26] . Matriptase is exclusively expressed in the epithelial cells in normal mammary glands and in the cancer cells of MMTV-PymT oncogene-induced carcinomas with no detectable expression in the stroma ( Fig. 1a ). Matriptase protein is detected in normal primary cells at low levels, and the expression is increased in mammary carcinoma cells as determined by western blotting ( Fig. 1b ). Furthermore, matriptase is present in its proteolytically active form in mammary epithelial cells, and the level of active matriptase is significantly increased in mammary carcinoma cells in comparison to normal mammary epithelial cells, as demonstrated by gelatin zymography ( Fig. 1b ). Importantly, the findings that matriptase is specifically expressed in the epithelial compartment and upregulated during carcinogenesis is in accordance with previous findings in human breast carcinomas rendering this tumour model particularly well-suited to understand the role of matriptase in tumour progression in humans [3] , [5] . 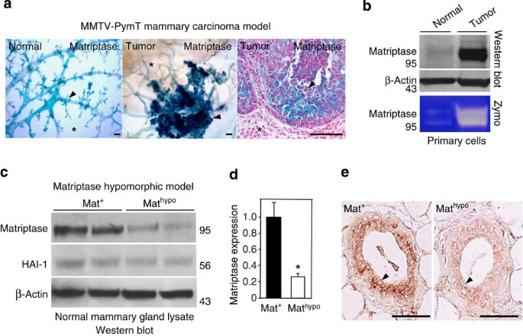Figure 1: Expression of matriptase in the MMTV-PymT mammary carcinoma model and matriptase hypomorphic model. (a) A knock-in mouse with a promoterless β-galactosidase marker gene inserted into the endogenous matriptase gene was used for precise assessment of endogenous matriptase expression in the mammary gland by X-gal staining (blue colour). Matriptase is expressed in the mammary gland epithelium (arrowhead ina) with no detectable expression in the stroma (*) in whole mounts from normal glands (left panel) and MMTV-PymT-induced carcinomas (middle panel). Histological analysis shows matriptase expression in the mammary cancer cells of MMTV-PymT transgenic mice (arrowhead, right panel). (b) Mammary epithelial cells from normal glands and tumour-bearing glands were isolated and analysed by western blotting (top panel) and gelatin zymography (lower panel) demonstrating increased levels of active matriptase in mammary carcinoma cells. (c) Western blot analysis of whole mammary gland extracts from matriptase hypomorphic mice (Mathypo) and control (Mat+) littermates with anti-matriptase (upper panel) or anti-HAI-1 (middle panel) antibodies. The levels of matriptase are greatly reduced in the Mathypomice. Importantly, levels of the epithelia-specific, physiological matriptase inhibitor, HAI-1, are comparable in Mathypoand Mat+glands. (d) Relative matriptase expression in Mathypomice (N=3) and Mat+mice (N=3) was determined by densitometry. Matriptase levels were normalized to HAI-1. Error bars represent s.d.P<0.04, Student’st-test. (e) Immunohistochemical staining of mammary glands from virgin females with a sheep anti-matriptase antibody confirming that matriptase protein expression in the ductal epithelium is greatly reduced in the Mathypomice. Scale bars, 50 μm. Figure 1: Expression of matriptase in the MMTV-PymT mammary carcinoma model and matriptase hypomorphic model. ( a ) A knock-in mouse with a promoterless β-galactosidase marker gene inserted into the endogenous matriptase gene was used for precise assessment of endogenous matriptase expression in the mammary gland by X-gal staining (blue colour). Matriptase is expressed in the mammary gland epithelium (arrowhead in a ) with no detectable expression in the stroma (*) in whole mounts from normal glands (left panel) and MMTV-PymT-induced carcinomas (middle panel). Histological analysis shows matriptase expression in the mammary cancer cells of MMTV-PymT transgenic mice (arrowhead, right panel). ( b ) Mammary epithelial cells from normal glands and tumour-bearing glands were isolated and analysed by western blotting (top panel) and gelatin zymography (lower panel) demonstrating increased levels of active matriptase in mammary carcinoma cells. ( c ) Western blot analysis of whole mammary gland extracts from matriptase hypomorphic mice (Mat hypo ) and control (Mat + ) littermates with anti-matriptase (upper panel) or anti-HAI-1 (middle panel) antibodies. The levels of matriptase are greatly reduced in the Mat hypo mice. Importantly, levels of the epithelia-specific, physiological matriptase inhibitor, HAI-1, are comparable in Mat hypo and Mat + glands. ( d ) Relative matriptase expression in Mat hypo mice ( N =3) and Mat + mice ( N =3) was determined by densitometry. Matriptase levels were normalized to HAI-1. Error bars represent s.d. P <0.04, Student’s t -test. ( e ) Immunohistochemical staining of mammary glands from virgin females with a sheep anti-matriptase antibody confirming that matriptase protein expression in the ductal epithelium is greatly reduced in the Mat hypo mice. Scale bars, 50 μm. Full size image Reduced matriptase in hypomorphic mammary glands We have previously generated matriptase hypomorphic mice (Mat hypo ) harbouring one St14 null allele and one St14 ‘knockdown’ allele in which an engrailed-2 splice acceptor site had been inserted between coding exons 1 and 2 (refs 25 , 26 , 27 ). These mice display an 80–99% reduction in matriptase mRNA levels in different tissues and have normal postnatal and long-term survival [27] . To assess the level of matriptase protein in the mammary gland of Mat hypo mice, western blot analysis of protein lysates of whole glands was performed ( Fig. 1c ). The level of matriptase protein in the mammary gland in Mat hypo mice is reduced >75% ( Fig. 1d ) as compared with littermate control mice (Mat + ). Immunohistochemical staining of mammary glands also confirmed that matriptase protein expression in the ductal epithelium is greatly reduced in the Mat hypo mice ( Fig. 1e ). Importantly, the residual matriptase in the mammary gland suffices to sustain normal mammary gland development based on comparative morphological and histological assessment ( Supplementary Fig. 1a ). Furthermore, Mat hypo females have functional mammary epithelium as they are lactation competent, and no reduction in litter size or litter weights is observed ( Supplementary Fig. 1b ). Thus, this model is well-suited to study progression of breast cancer in morphologically and functionally normal mammary glands with greatly reduced levels of matriptase. Reduced matriptase impairs mammary carcinogenesis To investigate the effects of low matriptase levels in the mammary gland on mammary carcinoma progression, Mat hypo and Mat + mice harbouring the MMTV-PymT oncogene were generated (referred to as PymT-Mat hypo and PymT-Mat + mice, respectively). Prospective cohorts with littermate PymT-Mat hypo and PymT-Mat + virgin female mice were established and monitored by weekly palpation to determine the appearance of the first palpable mammary mass (tumour latency). At 145 days of age, the number of glands with visible and palpable tumours was recorded (tumour multiplicity) and the area of tumours was determined by caliper measurements. Total mammary tumour burden was calculated as the total weight of all post-mortem excised mammary glands in individual mice from a cohort of female littermates. Reduced levels of matriptase in the mammary glands had significant effects on all tumorigenic parameters measured ( Fig. 2 ). Thus, the total tumour burden was reduced by 58% and the tumour growth rate was reduced by 76% ( Fig. 2a,b ). Also, tumour multiplicity was reduced by 45% ( Fig. 2d ). These results demonstrate that matriptase is an important contributor to tumour growth and progression. Notably, there was a significant delay in initial formation of palpable mammary tumours, indicating that matriptase is critical for early carcinogenesis with a mean latency of palpable tumours of 84 days in PymT-Mat + mice versus 120 days in PymT-Mat hypo mice ( Fig. 2c ). At 90 days, 53% of PymT-Mat + mice had palpable tumours versus 21% of PymT-Mat hypo mice. To examine the role of matriptase in early mammary carcinogenesis in further detail, an independent cohort was established and dysplastic lesions in the inguinal mammary glands were examined postmortem by whole mount analysis at 90 days of age ( Fig. 2e ). Importantly, total area measurements of lesions revealed a 75% reduction in the glands from PymT-Mat hypo mice as compared with PymT-Mat + ( Fig. 2f ). Taken together, these data strongly support a functional role for matriptase in both tumour formation and tumour growth. 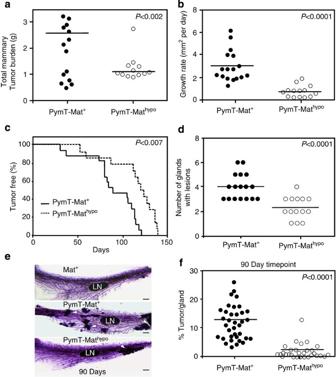Figure 2: Reduced matriptase decreases mammary tumour burden, growth rate, latency and multiplicity. A prospective cohort of littermate PymT-Mat+mice (N=14) and PymT Mathypomice (N=12) was followed over time. (a) Tumour burden at 145 days. Mice were euthanized and their mammary tumours resected and the total tumour weight was recorded for PymT Mat+mice (closed circles) and PymT-Mathypomice (open circles). Mean values were 2.6 and 1.1, respectively (P<0.002). (b) Mammary tumour growth rate for PymT-Mat+mice (closed circles) and PymT-Mathypomice (open circles). Mean values were 2.9 and 0.7, respectively (P<0.0001). (c) Kaplan–Meier tumour-free survival curves of PymT-Mat+(black line) and PymT-Mathypo(dotted line). The median tumour-free survival times were 89 days versus 122 days, respectively (P<0.007), chi-squared test. (d) Total number of glands with lesions at 145 days for PymT- Mat+mice (closed circles) and PymT-Mathypomice (open circles). Mean values were 4.0 and 2.2, respectively (P<0.0001). (e) Representative whole mounts of inguinal mammary glands from 90-day-old virgin female littermates. Normal mammary epithelium in Mat+gland (upper panel), extensive growth of multiple lesions (arrowheads) in PymT-Mat+gland (middle panel) and one small localized lesion (arrowhead) in PymT-Mathypogland (lower panel). LN=lymph node. (f) Total area of lesions in inguinal mammary glands from PymT-Mat+(closed circles) and PymT-Mathypo(open circles) (P<0.0001). Mann–WhitneyU-test was used ina,b,dandf. Scale bars, 1 mm. Figure 2: Reduced matriptase decreases mammary tumour burden, growth rate, latency and multiplicity. A prospective cohort of littermate PymT-Mat + mice ( N =14) and PymT Mat hypo mice ( N =12) was followed over time. ( a ) Tumour burden at 145 days. Mice were euthanized and their mammary tumours resected and the total tumour weight was recorded for PymT Mat + mice (closed circles) and PymT-Mat hypo mice (open circles). Mean values were 2.6 and 1.1, respectively ( P <0.002). ( b ) Mammary tumour growth rate for PymT-Mat + mice (closed circles) and PymT-Mat hypo mice (open circles). Mean values were 2.9 and 0.7, respectively ( P <0.0001). ( c ) Kaplan–Meier tumour-free survival curves of PymT-Mat + (black line) and PymT-Mat hypo (dotted line). The median tumour-free survival times were 89 days versus 122 days, respectively ( P <0.007), chi-squared test. ( d ) Total number of glands with lesions at 145 days for PymT- Mat + mice (closed circles) and PymT-Mat hypo mice (open circles). Mean values were 4.0 and 2.2, respectively ( P <0.0001). ( e ) Representative whole mounts of inguinal mammary glands from 90-day-old virgin female littermates. Normal mammary epithelium in Mat + gland (upper panel), extensive growth of multiple lesions (arrowheads) in PymT-Mat + gland (middle panel) and one small localized lesion (arrowhead) in PymT-Mat hypo gland (lower panel). LN=lymph node. ( f ) Total area of lesions in inguinal mammary glands from PymT-Mat + (closed circles) and PymT-Mat hypo (open circles) ( P <0.0001). Mann–Whitney U -test was used in a , b , d and f . Scale bars, 1 mm. Full size image Reduced matriptase impairs tumour proliferation The cause of mammary tumour growth attenuation in mice with low matriptase was addressed through analysis of proliferation, macrophage infiltration and apoptosis ( Fig. 3 ). Proliferation rates of carcinoma cells were determined at two different time points by immunohistochemical detection of bromodeoxyuridine (BrdU) or endogenous Ki67 ( Fig. 3 ). At 127 days of age, carcinoma cell proliferation was reduced by 47% in PymT-Mat hypo mice as compared with PymT-Mat + mice ( Fig. 3a,b ). A dramatic decrease in proliferation was also observed in PymT-Mat hypo 145-day-old mice with an 81% reduction as compared with littermate PymT-Mat + mice ( Fig. 3c ). No significant difference in tumour infiltration by macrophages, as determined by F4/80 staining, was detected ( Fig. 3d,f ), and the percentage of apoptotic cells visualized by terminal deoxynucleotidyl transferase (TdT)-mediated dUTP nick end labelling (TUNEL) staining was not significantly different ( Fig. 3e,g ). These data strongly suggest that matriptase-dependent carcinoma cell proliferation promotes mammary tumour growth and that the decrease in proliferative mammary carcinoma cells observed in PymT-Mat hypo mice is a major contributing factor to the abrogation of primary tumour growth. 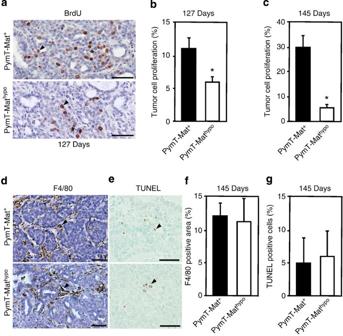Figure 3: Decreased carcinoma cell proliferation in mammary tumours with reduced matriptase. (a) Representative pictures of mammary tumours from PymT-Mat+(top) and PymT-Mathypo(bottom) stained with an anti-BrdU antibody. Mice were injected with BrdU 2 h before euthanasia. (b) Quantification of carcinoma cell proliferation in 127-day-old mice. Data are presented as the mean relative number of cells with positive nuclear BrdU staining (arrowheads) in tumours from PymT-Mat+(N=4, black bar), and littermate PymT-Mathypomice (N=3, white bar). (c) Quantification of carcinoma cell proliferation in 145-day-old mice. Data are presented as the mean relative number of cells with positive nuclear Ki67 staining in tumours from PymT-Mat+(N=4, black bar), and littermate PymT-Mathypomice (N=4, white bar). (d) Tumour-associated macrophages in 145-day-old mice. Macrophages were visualized using a rabbit anti-F4/80 antibody (arrowheads). (e) Apoptotic carcinoma cells detected by TUNEL staining in 145-day-old mice (arrowheads). (f) Quantification of tumour-associated macrophages. Data are presented as the mean relative area with positive F4/80 staining in tumours from PymT-Mat+(N=4, black bar), and littermate PymT-Mathypomice (N=3, white bar). (g) Quantification of cells with TUNEL-positive nuclear staining in tumours from PymT-Mat+(N=4, black bars), and littermate PymT-Mathypomice (N=3, white bars). All panels: Error bars represent s.d., *P<0.001, Mann–WhitneyU-test. Scale bars, 50 μm. Figure 3: Decreased carcinoma cell proliferation in mammary tumours with reduced matriptase. ( a ) Representative pictures of mammary tumours from PymT-Mat + (top) and PymT-Mat hypo (bottom) stained with an anti-BrdU antibody. Mice were injected with BrdU 2 h before euthanasia. ( b ) Quantification of carcinoma cell proliferation in 127-day-old mice. Data are presented as the mean relative number of cells with positive nuclear BrdU staining (arrowheads) in tumours from PymT-Mat + ( N =4, black bar), and littermate PymT-Mat hypo mice ( N =3, white bar). ( c ) Quantification of carcinoma cell proliferation in 145-day-old mice. Data are presented as the mean relative number of cells with positive nuclear Ki67 staining in tumours from PymT-Mat + ( N =4, black bar), and littermate PymT-Mat hypo mice ( N =4, white bar). ( d ) Tumour-associated macrophages in 145-day-old mice. Macrophages were visualized using a rabbit anti-F4/80 antibody (arrowheads). ( e ) Apoptotic carcinoma cells detected by TUNEL staining in 145-day-old mice (arrowheads). ( f ) Quantification of tumour-associated macrophages. Data are presented as the mean relative area with positive F4/80 staining in tumours from PymT-Mat + ( N =4, black bar), and littermate PymT-Mat hypo mice ( N =3, white bar). ( g ) Quantification of cells with TUNEL-positive nuclear staining in tumours from PymT-Mat + ( N =4, black bars), and littermate PymT-Mat hypo mice ( N =3, white bars). All panels: Error bars represent s.d., * P <0.001, Mann–Whitney U -test. Scale bars, 50 μm. Full size image Genetic ablation of matriptase abolishes c-Met signalling To better understand the pathophysiological function of matriptase, its proteolytic targets need to be identified. Of the candidate substrates for matriptase that have been identified thus far, HGF has been shown to directly promote mammary carcinogenesis, and therefore, is of particular interest [28] , [29] . HGF is secreted in its inactive pro-form by stromal cells in both human and mice, including stromal mammary fibroblasts and macrophages [30] , [31] , [32] . To date, no mammary gland genetic matriptase loss-of-function studies have been published and it is unknown whether matriptase is critical for pro-HGF activation and c-Met signalling in mammary cancer. For our studies, we used MMTV-PymT-induced primary mammary carcinoma cells from conditional matriptase knock-out mice (PymT-Mat cond.ko ) carrying a ubiquitously expressed inducible Cre recombinase fused to a mutated human estrogen receptor (Cre-ER), which allows for permanent inactivation of floxed matriptase alleles upon brief exposure to 4-hydroxy-tamoxifen (4-OHT) [33] , [34] . As shown in Fig. 4a , efficient matriptase ablation was induced ex vivo in PymT-Mat cond.ko mammary carcinoma and confirmed by western blot analysis. Exposure to serum-free media conditioned with fibroblast-secreted pro-HGF [35] caused robust c-Met activation in PymT-Mat control cells, as determined by phosphorylated c-Met (p-c-Met) protein levels ( Fig. 4b ). Activation of the two downstream cytoplasmic effector proteins, Gab1 and AKT, was also observed. In contrast, in PymT-Mat cond.ko mammary carcinoma cells, activation of c-Met, Gab1 and AKT was efficiently abrogated. Importantly, stimulation of matriptase-deficient cells with pre-cleaved two-chain active HGF did not affect phosphorylation of c-Met, Gab1 or AKT ( Fig. 4b ). This demonstrates that the effects of matriptase gene ablation on cell signalling is caused by the loss of matriptase-mediated proteolytic conversion of inactive pro-HGF to active HGF, and thereby, its ability to initiate the c-Met signalling pathway. Also, PymT-Mat cond.ko cells retain the ability to cleave pro-HGF and activate c-Met signalling following treatment with vehicle instead of the Cre-ER recombination-inducing agent, 4-OHT ( Supplementary Fig. 2 ). 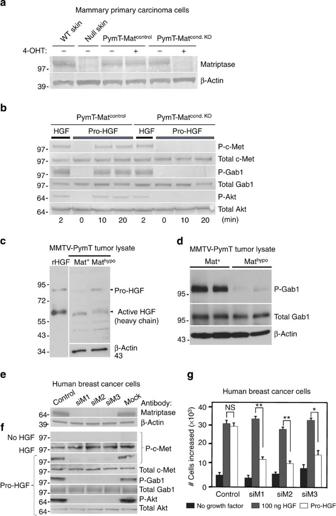Figure 4: Matriptase is required for activation of the pro-HGF/c-Met signalling pathway and cell proliferation in primary mammary carcinoma cells, mammary tumours and human breast cancer cells. (a) Efficient Cre-mediated ablation of matriptase in primary mammary carcinoma cells shown by western blot analysis of cells isolated from PymT-Matcond KOor PymT-Matcontrolmice. Two days after plating, 10 μM 4-OHT (+) or vehicle (−) was added 24 h to ablate matriptase expression. Cells were in serum-free medium without 4-OHT for another 24 h before lysis. Skin lysates from newborn matriptase null and wild-type littermate mouse were included for antibody specificity. Anti-β-actin was used as control for equal loading. (b) Mammary carcinoma cells were isolated and treated with 4-OHT as above and exposed to active HGF (2 min) or pro-HGF (0, 10 or 20 min). Cell lysates were analysed for total c-Met, activated c-Met and its downstream targets by western blotting. (c,d) Whole lysates of mammary tumours were separated by reducing SDS–PAGE and analysed by western blotting. (c) HGF is mainly present in its active two-chain form in PymT-Mat+tumours, whereas a significant level of single-chain, inactive pro-HGF is detected in PymT-Mathypotumours. rHGF=recombinant pro-HGF/HGF. (d) reduced Gab1 levels of the active phosphorylated form relative to total Gab1 in PymT-Mathypomammary tumours. (e) Efficient RNAi silencing of matriptase in human HCC1937 cells with three non-overlapping synthetic RNA duplexes (siM1, siM2 and siM3). A %GC matched RNA duplex was used as negative control as well as a mock (no RNA duplex). β-Actin staining ensured equal protein loading. (f) Cells were serum staved and exposed to no HGF, active HGF (2 min) or pro-HGF (15 min). Lysates were analysed for total c-Met, activated c-Met and its downstream targets. (g) Matriptase was silenced in HCC1937 cells as above and left untreated (black bars) or exposed to active HGF (grey bars) or pro-HGF (white bars) for 24 h. Bar graphs show proliferation 24 h after stimulation (*P<0.04, **P<0.005, ***P<0.0008, Student’st-test). Data represent mean of three replicates. Error bars represent s.d. Data are representative of four independent experiments. Figure 4: Matriptase is required for activation of the pro-HGF/c-Met signalling pathway and cell proliferation in primary mammary carcinoma cells, mammary tumours and human breast cancer cells. ( a ) Efficient Cre-mediated ablation of matriptase in primary mammary carcinoma cells shown by western blot analysis of cells isolated from PymT-Mat cond KO or PymT-Mat control mice. Two days after plating, 10 μM 4-OHT (+) or vehicle (−) was added 24 h to ablate matriptase expression. Cells were in serum-free medium without 4-OHT for another 24 h before lysis. Skin lysates from newborn matriptase null and wild-type littermate mouse were included for antibody specificity. Anti-β-actin was used as control for equal loading. ( b ) Mammary carcinoma cells were isolated and treated with 4-OHT as above and exposed to active HGF (2 min) or pro-HGF (0, 10 or 20 min). Cell lysates were analysed for total c-Met, activated c-Met and its downstream targets by western blotting. ( c , d ) Whole lysates of mammary tumours were separated by reducing SDS–PAGE and analysed by western blotting. ( c ) HGF is mainly present in its active two-chain form in PymT-Mat + tumours, whereas a significant level of single-chain, inactive pro-HGF is detected in PymT-Mat hypo tumours. rHGF=recombinant pro-HGF/HGF. ( d ) reduced Gab1 levels of the active phosphorylated form relative to total Gab1 in PymT-Mat hypo mammary tumours. ( e ) Efficient RNAi silencing of matriptase in human HCC1937 cells with three non-overlapping synthetic RNA duplexes (siM1, siM2 and siM3). A %GC matched RNA duplex was used as negative control as well as a mock (no RNA duplex). β-Actin staining ensured equal protein loading. ( f ) Cells were serum staved and exposed to no HGF, active HGF (2 min) or pro-HGF (15 min). Lysates were analysed for total c-Met, activated c-Met and its downstream targets. ( g ) Matriptase was silenced in HCC1937 cells as above and left untreated (black bars) or exposed to active HGF (grey bars) or pro-HGF (white bars) for 24 h. Bar graphs show proliferation 24 h after stimulation (* P <0.04, ** P <0.005, *** P <0.0008, Student’s t -test). Data represent mean of three replicates. Error bars represent s.d. Data are representative of four independent experiments. Full size image To assess whether the matriptase-mediated activation of the HGF/c-Met signalling pathway observed in primary mammary tumour cells is relevant in whole tumours, the activation state of HGF in tumour extracts was determined in PymT-Mat hypo and PymT-Mat + mice. HGF is detected mainly in its active form in matriptase control tumours, whereas a significant fraction (approximately 50–80%) of the growth factor is present in its non-cleaved, single-chain, pro-form in tumours from matriptase hypomorphic mice ( Fig. 4c ). To further elucidate whether the reduced levels of active HGF lead to decreased activation of the c-Met signalling pathway, the levels of p-Gab1 in whole tumour lysates were analysed. Gab-1 is a docking protein that binds the phosphorylated c-Met receptor tyrosine kinase directly and mediates c-Met signalling. The essential role of Gab1 for signalling by the c-Met receptor has been demonstrated in vivo [36] . A pronounced decrease in P-Gab1 expression in tumours from matriptase hypomorphic mice as compared with control mice was observed, whereas the levels of total Gab1 proteins were not affected ( Fig. 4d ). Taken together, these data suggest that matriptase-mediated proteolytic conversion of pro-HGF to active HGF is critical for activation of the c-Met signalling pathway, and that decreased levels of matriptase cause abated activation of the c-Met-mediated signalling and proliferation in vivo . Matriptase-mediated proliferation in human breast cancer To verify the relevance of matriptase-dependent pro-HGF activation in human breast cancer, we used three different human breast cancer cell lines of diverse origin: BT20, SUM229 and HCC1937, which were confirmed to express matriptase and c-Met ( Figs 4e,f and Supplementary Fig. 3a, a′,b,b′ ). Matriptase was efficiently silenced in all three human breast cancer cell lines using three independent, non-overlapping synthetic RNA duplexes. Addition of pro-HGF to HCC1937 matriptase-sufficient control cells resulted in robust activation of c-Met and the downstream targets, Gab1 and Akt ( Fig. 4f ). In contrast, matriptase ablation led to a greatly reduced level of c-Met pathway activation rendering the phosphorylated forms of c-Met, Gab1 and Akt undetectable by western blotting. Importantly, the matriptase-silenced cells displayed unaltered activation of the c-Met pathway upon stimulation with pre-cleaved, active HGF, demonstrating that the matriptase-deficient cells have a fully functional c-Met signalling pathway, and that the impaired response to pro-HGF is due to the lack of the matriptase-mediated activation cleavage ( Fig. 4f ). Similar results for BT20 and SUM229 cells upon matriptase silencing were observed including efficient abrogation of the activation of c-Met, Gab1 and Akt ( Supplementary Fig. 3a ′ ,b′ ). This indicates that the mechanism observed is not limited to one cell line and may represent a general phenomenon in human breast cancer. Matriptase, in addition to being an efficient activator of pro-HGF, has been shown to cleave and activate the pro-form of urokinase-type plasminogen activator (pro-uPA) [28] , [29] , [37] , [38] . Furthermore, it has been demonstrated that active uPA itself can cleave and activate pro-HGF in vitro [39] , [40] , [41] . To test whether uPA plays a role in activation of pro-HGF in breast cancer cells, silencing of uPA was performed ( Supplementary Fig. 4a ). RNAi-mediated uPA knockdown did not result in any discernable changes in c-Met activation upon stimulation with pro-HGF, indicating that matriptase directly cleaves and activates the growth factor in a uPA-independent manner in breast cancer cells ( Supplementary Fig. 4b ). Also, the status of uPA activation in mammary tumours was assessed by reducing western blot analysis using whole tissue lysates of tumours from matriptase hypomorphic mice and control mice. uPA is present in both its single-chain pro-form and two-chain active form in mammary tumours and no discernible differences in the pro-uPA/active uPA ratio were observed between PymT-Mat + and PymT-Mat hypo tumours ( Supplementary Fig. 4c ). This suggests that matriptase is not a critical activator of pro-uPA in breast cancer in the in vivo model used in this study. To assess the functional consequences of inhibiting the matriptase-meditated HGF/c-Met signalling in human breast cancer cells, we assessed proliferation in the matriptase-silenced BT20, HCC1937 and SUM229 cell lines. Following matriptase silencing in cells with three different synthetic RNA duplexes, cells were treated with pro-HGF or active pre-cleaved HGF and proliferation during 24 h was determined ( Fig. 4g and Supplementary Fig. 3 ). As expected, there was no significant proliferation difference in matriptase-sufficient HCC1937 cells treated with either active HGF or pro-HGF. In contrast, the proliferation in matriptase-silenced cells was significantly impaired in response to pro-HGF in comparison to the response observed in HGF-treated cells ( Fig. 4g ). Similar results were obtained with the SUM229 and BT20 cell lines ( Supplementary Fig. 3a ′′ ,b ′′ ). These results demonstrate that silencing matriptase leads to decreased pro-HGF activation and subsequent c-Met signalling pathway activation, ultimately causing growth inhibition. In addition, a ‘gain-of-function’ experiment using SUM159 cells that have lost the expression of endogenous matriptase and are non-responsive to pro-HGF was performed ( Supplementary Fig. 5 ). In spite of the loss of matriptase activity, SUM159 cells have retained the proliferation response capability upon stimulation with two-chain active HGF. Therefore, to investigate whether re-expression of matriptase could restore the ability of these cells to respond to pro-HGF, SUM159 cells were transiently transfected with a mammalian expression vector containing human full-length matriptase. Indeed, matriptase re-expression fully restored c-Met signalling in SUM159 human breast cancer cells in response to pro-HGF. The matriptase-mediated ability to activate the c-Met signalling pathway was accompanied by a strong mitogenic response to pro-HGF ( Supplementary Fig. 5c ). Taken together, by performing ‘loss-of-function’ studies for mouse mammary carcinoma cells, mouse mammary tumours and human cancer cells, we have demonstrated that matriptase is a major activator of pro-HGF in model systems using either primary mammary carcinoma cells or three different established breast carcinoma cell lines. This conclusion is supported by the fact that no apparent compensation by one or more proteases, upon genetic ablation or post-transcriptional silencing of matriptase, was detected. Furthermore, the ‘gain-of-function’ study demonstrates that matriptase confers SUM159 breast cancer cells with the capability to activate pro-HGF, and thereby elicit the c-Met signalling pathway and subsequent proliferative response. Matriptase mediates invasion in human breast cancer cells Many cancer cell lines form spontaneous, three-dimensional (3D), multicellular, tumour-like spheroids when cultured in reconstituted basement membrane (rBM) overlay culture. These spheroids often resemble solid tumours, and tumorigenic processes including invasive growth, can therefore be studied in this model. HGF has been shown to induce invasiveness in a variety of cancer cells in 3D culture. When SUM229 cells were grown in rBM overlay culture, they spontaneously formed spheroids ( Fig. 5a,b ). Upon stimulation with pro-HGF for 24 h, matriptase-sufficient control cells displayed pronounced invasive growth characterized by branching, multicellular structures and single cells with a flattened spindle-like appearance ( Fig. 5a ′ ). Matriptase silencing in SUM229 spheroids (Mat KD) rendered the cells unresponsive to pro-HGF, thus, keeping the vast majority of the cells confined in compact spheroid structures ( Fig. 5b ′ and Supplementary Fig. 6 ). Addition of pre-cleaved active HGF restored the ability of matriptase-deficient cells to respond to the growth factor. These data demonstrate that matriptase, in addition to promoting breast cancer cell proliferation as described above, potentiates the invasive capacity of cancer cells, suggesting that matriptase-mediated c-Met signalling is critical for several pro-tumorigenic processes. 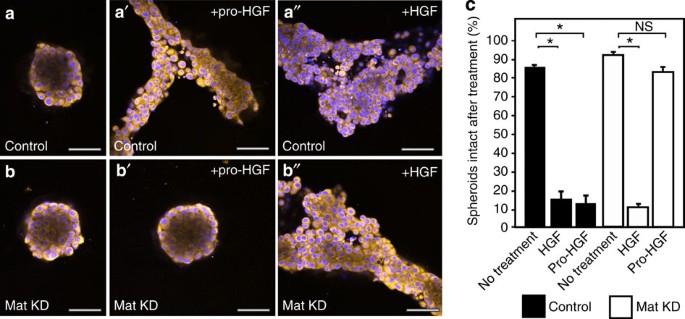Figure 5: Matriptase mediates pro-HGF-induced invasion in human breast cancer cells. SUM229 cells were grown on culture plates and matriptase was silenced (Mat KD) using synthetic RNA duplexes (b,b′,b′′). A %GC matched RNA duplex was used as negative control (a,a′,a′′). Cells were allowed to form spheroids in 3D rBM overlay culture for 24 h before addition of either pro-HGF (a′,b′), HGF (a′′,b′′) or no growth factors (a,b) and imaged by confocal microscopy. When no growth factors were added, control and Mat KD spheroids remained intact. In contrast, addition of pro-HGF-induced extensive invasive outgrowths in matriptase-sufficient control cells (a′), whereas the majority of Mat KD spheroids remained intact (b′). Both control and Mat KD spheroids responded to active two-chain HGF (a′′,b′′). Cells were labelled with Cell Tracker Orange and nuclei with Hoechst (blue). (c) 3D rBM cell cultures were scored for the number of intact spheroids when left untreated (black bars) or exposed to either active HGF (white bars) or pro-HGF (white bars). Data represent mean of the number of intact spheroids before treatment relative to the number after treatment (triplicates; *P<0.04, Student’st-test). Error bars represent s.d. Scale bars, 50 μm. Data are representative of four independent experiments. Figure 5: Matriptase mediates pro-HGF-induced invasion in human breast cancer cells. SUM229 cells were grown on culture plates and matriptase was silenced (Mat KD) using synthetic RNA duplexes ( b , b′ , b′′ ). A %GC matched RNA duplex was used as negative control ( a , a′ , a′′ ). Cells were allowed to form spheroids in 3D rBM overlay culture for 24 h before addition of either pro-HGF ( a′ , b′ ), HGF ( a′′ , b′′ ) or no growth factors ( a , b ) and imaged by confocal microscopy. When no growth factors were added, control and Mat KD spheroids remained intact. In contrast, addition of pro-HGF-induced extensive invasive outgrowths in matriptase-sufficient control cells ( a′ ), whereas the majority of Mat KD spheroids remained intact ( b′ ). Both control and Mat KD spheroids responded to active two-chain HGF ( a′′ , b′′ ). Cells were labelled with Cell Tracker Orange and nuclei with Hoechst (blue). ( c ) 3D rBM cell cultures were scored for the number of intact spheroids when left untreated (black bars) or exposed to either active HGF (white bars) or pro-HGF (white bars). Data represent mean of the number of intact spheroids before treatment relative to the number after treatment (triplicates; * P <0.04, Student’s t -test). Error bars represent s.d. Scale bars, 50 μm. Data are representative of four independent experiments. Full size image Correlated matriptase and c-Met expression in breast cancer To investigate whether the functional link identified between matriptase and c-Met is likely to represent a general molecular pro-tumorigenic mechanism in human breast cancer, the expression of matriptase and c-Met in a large sample set of 153 human invasive ductal carcinoma tumour tissues was analysed by immunohistochemistry ( Fig. 6 ). To ensure specific staining, two different antibodies raised against matriptase and c-Met, respectively, were used. An antibody recognizing p-c-Met was also included. The staining of invasive ductal carcinomas was strong and uniform for matriptase and c-Met in the cancer cells. Furthermore, the staining patterns observed for matriptase, c-Met and p-c-Met were strikingly similar, consistent with co-localization of the protease and the growth factor receptor (total and phosphorylated c-Met) in breast carcinomas ( Fig. 6a,c ). No significant staining was observed in tumour stromal compartments. The vast majority of tumour samples, 88% (134/153), displayed detectable expression of both matriptase and c-Met protein ( Fig. 6b ). A small subset of tumours, 7% (11/153), displayed no detectable expression of either matriptase or c-Met, whereas 5% (7/153) of the breast tumours expressed matriptase, but not c-Met. In only 0.7% (1/153) of the tumours, c-Met, but not matriptase protein, was detected. The overall comparison of groups showed a highly significant correlation between matriptase and c-Met expression in breast cancer. Importantly, co-expression of matriptase and c-Met was also consistently observed in MMTV-PymT tumours, further validating this breast tumour model as being highly relevant for studying the matriptase/pro-HGF/c-Met signalling axis ( Supplementary Fig. 7 ). 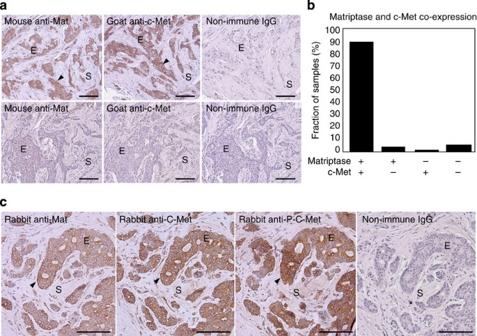Figure 6: Matriptase and c-Met expression are correlated in human invasive ductal carcinomas. Representative staining of serial sections of invasive ductal carcinoma (a) using a mouse monoclonal anti-matriptase antibody and a goat anti-c-Met antibody. Upper panels: carcinoma with matriptase and c-Met co-expression. Lower panels: carcinoma negative for both matriptase and c-Met. Primary antibodies were substituted with non-immune control IgG as negative controls. (b) Expression of matriptase and c-Met in 153 human invasive ductal carcinomas. Bars depict the frequency of samples expressing matriptase and c-Met (134/153), samples that express neither matriptase nor c-Met (11/153), samples that express only matriptase (7/153) and samples that express c-Met only as indicated (1/153). The overall comparison of groups showed a highly significant correlation between c-Met and matriptase expression: Tetrachoric Rho=0.95 (P<0.001). (c) Representative staining of serial sections of invasive ductal carcinoma using rabbit anti-matriptase, rabbit anti-c-Met and rabbit anti-phospho-c-Met. Matriptase, c-Met and phospho-c-Met (brown staining, arrow heads) are detected in the epithelia-derived cancer cells (indicated with ‘E’) with no significant staining in the mesenchymal/stromal compartments (indicated with ‘S’). Tissues were counterstained with haematoxylin (blue/grey). Both matriptase and c-Met are primarily localized on cell surfaces and in the cytoplasm and display highly similar expression patterns. Scale bars, 100 μm. Figure 6: Matriptase and c-Met expression are correlated in human invasive ductal carcinomas. Representative staining of serial sections of invasive ductal carcinoma ( a ) using a mouse monoclonal anti-matriptase antibody and a goat anti-c-Met antibody. Upper panels: carcinoma with matriptase and c-Met co-expression. Lower panels: carcinoma negative for both matriptase and c-Met. Primary antibodies were substituted with non-immune control IgG as negative controls. ( b ) Expression of matriptase and c-Met in 153 human invasive ductal carcinomas. Bars depict the frequency of samples expressing matriptase and c-Met (134/153), samples that express neither matriptase nor c-Met (11/153), samples that express only matriptase (7/153) and samples that express c-Met only as indicated (1/153). The overall comparison of groups showed a highly significant correlation between c-Met and matriptase expression: Tetrachoric Rho=0.95 ( P <0.001). ( c ) Representative staining of serial sections of invasive ductal carcinoma using rabbit anti-matriptase, rabbit anti-c-Met and rabbit anti-phospho-c-Met. Matriptase, c-Met and phospho-c-Met (brown staining, arrow heads) are detected in the epithelia-derived cancer cells (indicated with ‘E’) with no significant staining in the mesenchymal/stromal compartments (indicated with ‘S’). Tissues were counterstained with haematoxylin (blue/grey). Both matriptase and c-Met are primarily localized on cell surfaces and in the cytoplasm and display highly similar expression patterns. Scale bars, 100 μm. Full size image The finding that matriptase and c-Met are both expressed in the vast majority of the human invasive ductal carcinomas analysed, presents the opportunity for potential therapeutic intervention in a large number of breast cancer patients. Targeting matriptase proteolytic activity in breast cancer Based on our findings that matriptase is critically involved in breast cancer cell proliferation and invasion, and in tumour progression and growth, in vivo, this protease represents a promising target for drug development. To determine whether inhibition of matriptase proteolytic activity leads to abrogation of the c-Met signalling activation, we initially tested three matriptase inhibitors in murine and human breast cancer cell culture models. Leupeptin is a small peptide, reversible protease inhibitor with a broad spectrum of protease targets. HAI-1 and 2 are reversible, competitive, macromolecular Kunitz-type serine-protease inhibitors that have been shown to be physiological inhibitors of matriptase [42] , [43] , [44] , [45] . Leupeptin, HAI-1 and -2 efficiently inhibited c-Met activation upon pro-HGF stimulation in the three human breast cancer cell lines, BT20, HCC1937 and SUM229 ( Fig. 7a and Supplementary Fig. 8a ). None of the three inhibitors affected c-Met activation upon stimulation with pre-cleaved active HGF. To further investigate whether matriptase may represent a novel target for pharmaceutical intervention in breast cancer, the inhibitor of matriptase containing a ketobenzothiazole serine trap, IN-1, was tested [46] , [47] . IN-1 inhibited c-Met activation in both primary mammary carcinoma cells and in the three human breast cancer cell lines BT20, HCC1937 and SUM229 ( Fig. 7b and Supplementary Fig. 8b ). Notably, IN-1 inhibited pro-HGF-driven proliferation in all three human cell lines in a dose-dependent manner ( Fig. 7c and Supplementary Fig. 8c ). The inhibitory effect observed at 10 μM, 1 μM and as low as 100 nM was so efficient that the proliferation was abrogated to a level that was statistically indistinguishable from the level observed when no growth factor was added ( P >0.1). In sum, the development of selective and efficient inhibitors of matriptase proteolytic activity represents a potential new avenue for targeting the pro-tumorigenic c-Met signalling pathway by inhibition of the matriptase-dependent conversion of the signalling-inert single-chain, pro-HGF to a signalling-competent, two-chain HGF. 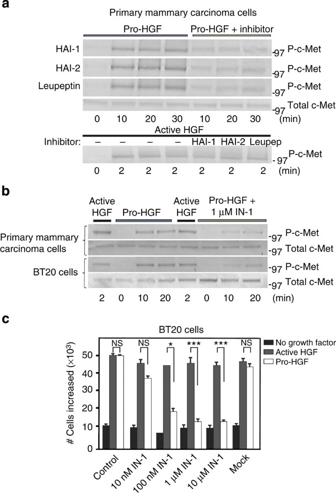Figure 7: Abrogation of pro-HGF-mediated c-met activation and breast cancer cell proliferation using matriptase inhibitors. (a) Matriptase-sufficient mouse mammary carcinoma cells were isolated from Mat-PymT+mice and exposed to pro-HGF or pre-cleaved active HGF with and without matriptase inhibitors added concomitantly (60 nM HAI-1, 40 nM HAI-2 or 20 μM leupeptin). Cells were lysed at the indicated time points after growth factor stimulation and analysed for total and activated c-Met by western blotting. (b) Mouse mammary carcinoma cells or human breast cancer BT20 cells were serum starved and pre-incubated with 1 μM IN-1 synthetic matriptase inhibitor for 30 min before exposure to active HGF, pro-HGF or no growth factors. Cells were lysed at the indicated time points after growth factor stimulation and analysed for total and activated c-Met by western blotting. (c) BT20 cells were serum starved and exposed to either active HGF (grey bars), pro-HGF (white bars) or no growth factor (black bars) for 24 h and counted. The synthetic selective matriptase inhibitor IN-1 was added at 10 nM, 100 nM, 1 μM or 10 μM concomitantly with pro-HGF/HGF. In the mock, control vehicle (PBS) was added. Graphs show the increase in cell numbers at 24 h after stimulation (triplicates; *P<0.04, **P<0.005, ***P<0.0008, Student’st-test). Error bars represent s.d. All data are representative of three independent experiments. Figure 7: Abrogation of pro-HGF-mediated c-met activation and breast cancer cell proliferation using matriptase inhibitors. ( a ) Matriptase-sufficient mouse mammary carcinoma cells were isolated from Mat-PymT + mice and exposed to pro-HGF or pre-cleaved active HGF with and without matriptase inhibitors added concomitantly (60 nM HAI-1, 40 nM HAI-2 or 20 μM leupeptin). Cells were lysed at the indicated time points after growth factor stimulation and analysed for total and activated c-Met by western blotting. ( b ) Mouse mammary carcinoma cells or human breast cancer BT20 cells were serum starved and pre-incubated with 1 μM IN-1 synthetic matriptase inhibitor for 30 min before exposure to active HGF, pro-HGF or no growth factors. Cells were lysed at the indicated time points after growth factor stimulation and analysed for total and activated c-Met by western blotting. ( c ) BT20 cells were serum starved and exposed to either active HGF (grey bars), pro-HGF (white bars) or no growth factor (black bars) for 24 h and counted. The synthetic selective matriptase inhibitor IN-1 was added at 10 nM, 100 nM, 1 μM or 10 μM concomitantly with pro-HGF/HGF. In the mock, control vehicle (PBS) was added. Graphs show the increase in cell numbers at 24 h after stimulation (triplicates; * P <0.04, ** P <0.005, *** P <0.0008, Student’s t -test). Error bars represent s.d. All data are representative of three independent experiments. Full size image Matriptase is an epithelial cell-surface protease that is highly expressed in human breast cancer. In this study, the specific functions of matriptase in mammary tumorigenesis were investigated by using a mouse model of human ductal mammary adenocarcinoma. Mice with low matriptase expression in the mammary epithelium displayed a significant delay in tumour onset, tumour burden and multiplicity. Notably, a significant abrogation of tumour progression was seen in early stages of carcinogenesis. A major factor contributing to tumour growth impairment was the dramatic decrease in carcinoma cell proliferation in matriptase hypomorphic tumours. To elucidate the molecular mechanisms underlying matriptase-mediated proliferation, we utilized an ex vivo model with primary mammary carcinoma cells, as well as 2D and 3D human breast cancer cell culture models. We demonstrate that matriptase is necessary to initiate the activation of the c-Met signalling pathway in response to fibroblast-secreted pro-HGF by cleaving and activating the growth factor. HGF is an important promoter of proliferation and invasion in cancer, and its receptor, c-Met, like matriptase, is expressed in the epithelial compartment of the breast. The inactive pro-form of HGF binds to the c-Met tyrosine kinase receptor where, upon proteolytic cleavage, it is converted to the signalling-competent active form of HGF. This HGF-mediated c-Met signalling activates multiple downstream targets, including the PI3/AKT pathway, and the c-Met docking protein, Gab1. Until now, the protease responsible for pro-HGF activation in breast cancer was unknown. Using matriptase-deficient primary mammary carcinoma cells, we demonstrate that matriptase is essential for activation of fibroblast-secreted pro-HGF and initiation of downstream c-Met signalling. The in vivo relevance was confirmed in tumours where the levels of activated phosho-Gab1 were decreased in tumours from matriptase hypomorphic mice. Furthermore, the amounts of active tumoural HGF were reduced in matriptase hypomorphic mice. The findings in mouse mammary cancer were verified in human breast cancer using matriptase silencing in three different cell lines, which lead to abrogation of c-Met, Gab1 and Akt activation upon pro-HGF stimulation. Furthermore, re-expression of matriptase rescued c-Met activation in a cell line that has lost endogenous matriptase expression, and rescued the capability to respond to pro-HGF. In addition, we demonstrate that the functional consequence of abrogating matriptase is severe impairment of HGF-driven proliferation and invasion in breast cancer. Matriptase-mediated pro-HGF activation and c-Met signalling in the breast cancer models used does not appear to be dependent on uPA. This is likely due to the fact that uPA has been shown to be at least four orders of magnitude less efficient than matriptase in activating pro-HGF [38] . In addition to using genetic ablation and post-transcriptional silencing of matriptase, we also employed inhibitors of matriptase catalytic activity. The small-molecule, selective matriptase inhibitor, IN-1, efficiently abrogated c-Met activation and blocked breast cancer cell proliferation. These data demonstrate that matriptase-mediated proteolytic activation of pro-HGF and c-Met signalling is critical in breast cancer and that targeting of matriptase proteolytic activity efficiently inhibits breast cancer cell proliferation via a mechanism conserved in mice and humans. As breast cancer cells express a variety of extracellular proteases, it is somewhat surprising that none of these appear to be capable of cleaving and activating pro-HGF in either mouse primary mammary carcinoma cells or human breast cancer cells, when matriptase expression is ablated. HGF activator (HGFA) has been reported to be expressed in multiple breast cancer cell lines and in human breast tumours [48] . It should be mentioned, however, that despite its name, no evidence has been presented that implicates HGFA as a physiological relevant pro-HGF activator. In genetic targeting studies in mice, both HGF null and c-Met null mice display an embryonic lethal phenotype, whereas HGFA-null mice develop normally to term and have no discernable phenotype in adult mice [49] , [50] , [51] . This suggests that HGFA is dispensable as a pro-HGF activator during development and postnatal life. Studies assessing the role of HGFA in tumorigenesis in vivo have not been published. Two other members of the type II transmembrane serine protease family, hepsin and TMPRSS13, which have previously been reported as being able to cleave and activate pro-HGF in vitro , were readily detectable by western blot analysis in a variety of breast cancer cells lines (unpublished data), which included the HCC1937, SUM229 and BT20 lines used in this study. Since no or minimal residual pro-HGF-activating activity was detected upon matriptase silencing, it is unlikely that these proteases act as efficient pro-HGF activators on the cell surface of breast cancer cells. It can be argued that acute matriptase ablation may not allow breast cancer cells time to mobilize compensatory mechanisms. Countering this possibility is the fact that the SUM159 cell line that has lost endogenous matriptase, which remains undetectable through several years and multiple passages, expresses high levels of both hepsin and TMPRSS13, yet requires transgenic re-expression of matriptase in order to respond to pro-HGF stimulation. Several possible scenarios could explain why matriptase is an efficient cellular pro-HGF activator. In in vitro experiments using recombinant soluble active forms of hepsin and matriptase, hepsin is approximately tenfold less efficient than matriptase in activating pro-HGF, whereas matriptase and HGFA display similar efficiency [38] . However, the level of active matriptase in comparison to active hepsin or active HGFA in breast cancer cells is not known. Also, matriptase is able to efficiently cleave pro-HGF on the cell surface [38] , which may give it an advantage over HGFA, a soluble protease, as activated HGF can be specifically generated at its site of action. It remains to be determined whether the membrane localization of matriptase provides the protease with a kinetic advantage and whether the stem-region domains are involved in substrate recognition or interaction with c-Met. Thus, factors including activation state, membrane-anchoring, localization in cell membrane microdomains and interaction between protease and c-Met could favour matriptase in certain cellular microenvironments, including breast cancer. It should be mentioned that it is plausible that other proteases contribute to pro-HGF activation in whole organisms (mice and human). Based on the data presented, further development and testing of selective matriptase inhibitors may represent a new avenue for targeted therapy in breast cancer. As demonstrated, matriptase is critically involved in the activation of c-Met-dependent pro-tumorigenic processes in vivo , ex vivo and in breast cancer cell lines. Importantly, the fact that matriptase and c-Met display strongly correlated expression patterns in human breast tumours, suggests that targeting the matriptase-mediated c-Met signalling cascade has the potential for broad clinical application. One factor to consider is the potential side-effects of matriptase inhibition in patients. Based on studies in mouse genetic models, the skin and the gastrointestinal tract would likely be the most sensitive tissues where matriptase-targeted drugs could cause adverse effects. However, hypomorphic mice, which have <1% residual epidermal and intestinal matriptase, display only a mild and temporary ichthyosis of the skin in very young mice, and a mild gut barrier defect with no discernible consequences for adult mouse health [52] , [53] . Furthermore, humans with a hypomorphic mutation in the St14 gene, resulting in a matriptase mutant protein with a 1,000-fold lower activity than that of wild-type matriptase, have a mild temporary ichthyosis of the skin and brittle hair that shows significant improvement with age. No gastrointestinal symptoms were reported [27] , [53] . It is therefore plausible that matriptase function in normal physiological processes in humans is predominantly critical during childhood, and that targeted inhibition in adults have few and mild adverse effects. In a recent article by the group of researchers that originally identified c-Met and characterized its biochemical properties, structure and function in development and disease, the rationale and progress of targeting c-Met in cancer is reviewed [22] . The c-Met inhibitors developed thus far include c-Met antagonists, such as antibodies that bind to c-Met and compete with pro-HGF/HGF binding, and c-Met kinase inhibitors. The authors mention targeting of pro-HGF-activating proteases as potential novel inhibitors of c-Met signalling and that resistance to kinase inhibitors may be circumvented by combining inhibitors with different modes of action. In conclusion, we demonstrate that matriptase is critical for breast carcinoma progression using multiple in vivo , ex vivo and cell culture approaches. Importantly, a mechanistic understanding of the pro-cancerous properties of matriptase has been reached by identifying matriptase as an essential activator of pro-HGF and initiator of the c-Met signalling pathway. The findings described here lay the foundation for future studies testing small-molecule matriptase inhibitors and their potential as novel targeted therapeutic drugs in breast cancer. Animals All procedures involving live animals were performed in an Association for Assessment and Accreditation of Laboratory Animal Care International-accredited vivarium following institutional guidelines and standard operating procedures. Generation of St14 hypomorphic mammary tumour mice Mice transgenic for the MMTV-Polyoma virus middle T oncogene ( PyVT ) in the FVB/N background (strain: FVB/N-Tg (MMTV-PyVT) 634Mul ) were obtained from The Jackson Laboratory and crossed with females carrying an St14 (matriptase) null allele ( St14 +/− ) [6] or an St14 knockdown/hypomorphic allele ( St14 +/hypo ) [27] in the C57BL/6 background. F1 PyVT/St14 +/− male pups were then mated to St14 +/hypo or ST14 hypo/hypo females to produce the study cohorts of F2 hypomorphic female mice carrying the PyVT transgene. PyVT/St14 −/hypo mice (referred to as: PymT-Mat hypo mice) and littermate control mice, PyVT/St14 +/+ , PyVT/St14 +/hypo or PyVT/St14 +/− (referred to as: PymT-Mat + mice. Genotyping of St14 wild-type, knockdown and null alleles was performed by PCR of ear or tail biopsy DNA [6] , [23] . Generation of St14 conditional knock-out mammary tumour mice The generation of the conditional matriptase knockout allele ( St14 LoxP ), as well as the St14 null allele carrying a β-galactosidase expression cassette ( St14 E16β-gal ), has been described previously [26] , [27] . Interbreeding of mice carrying these St14 alleles with mice carrying a 4-OHT-inducible Cre transgene (β- actin-Cre-ER tm +/0 mice, Strain: (B6.Cg-Tg(Cre/Esr1)5AMC/J) Jackson Laboratories) and FVB/N-Tg (MMTV-PyVT) 634Mul mice resulted in the generation of female (MMTV-PyVT) 634Mul /β- actin-Cre-ER tm +/00 ; St14 LoxP /E16β-gal study mice (referred to as PymT-Mat Cond. KO ) and their associated control littermates ( PyVT /β- actin-Cre-ER tm +/0 ; St14 LoxP /+ , PyVT/β- actin-Cre-ER tm +/0 ; St14 LoxP /E16β-gal , PyVT /β- actin-Cre-ER 0 ; St14 LoxP /E16β-gal , PyVT /β- actin-Cre-ER 0 ; St14 LoxP /+ (referred to as PymT-Mat + )). The genotypes of all mice were determined by PCR of ear or tail biopsy DNA [27] , [34] . Mammary gland whole mount analysis Mammary glands were fixed in Carnoy’s Fixative and stained in Carmine Alum. The area of cancerous lesions relative to the area of the entire mammary gland was determined with Image J (NIH software). Immunohistochemistry analysis of mouse tissue Tissues were fixed for 24 h in 10% neutral-buffered zinc formalin (Z-fix, Anatech), processed into paraffin and sectioned. Antigens were retrieved by heating in epitope retrieval buffer-reduced pH (Bethyl Laboratories). The sections were blocked for 1 h at room temperature with 3% bovine serum albumin in PBS and incubated overnight at 4 °C with primary antibody [34] . Primary antibodies used were sheep anti-matriptase (1:100) and goat anti-c-Met (1:100; R&D Systems). Cell proliferation was visualized by intraperitoneal injection of 100 μg g −1 BrdU (Sigma Chemical Co) 2 h before euthanasia. BrdU incorporation was detected with a rat anti-BrdU antibody (Accurate Chemical and Scientific Corporation, 1:10). Alternatively, a rabbit anti-Ki67 antibody (1:100; Thermo Scientific) was used. As negative controls, non-immune rabbit IgG, non-immune sheep IgG or non-immune goat IgG (Sigma) were used (adjusted to same final concentration as specific primary antibodies). Macrophages were detected by a rabbit anti-F4/80 antibody (1:100; Abcam). TUNEL was performed using a TACS 2 TdT-DAB In Situ Apoptosis Detection Kit (Trevigen) according to the manufacturer’s instructions. Breast cancer tissue array The use of human tissue paraffin-embedded samples was approved according to the Institutional Review Board Administration. The ‘BC20812’ and ‘BRC711’ breast cancer tissue arrays with pathology grading were obtained from US Biomax, Inc. Grade II and III tumours were analysed in this study. Tissue arrays were deparaffinized with xylene and hydrated with graded ethanol solutions. Antigen retrieval was performed using heated citrate buffer, reduced pH (Bethyl Laboratories). The arrays were blocked with 2% bovine serum albumin in PBS, and immunostained overnight at 4 °C (ref. 5 ). Primary antibodies were mouse anti-matriptase (1:200), goat anti-c-Met (1:200) and rabbit anti-phospho-cMet (1:200; R&D Systems), rabbit anti-matriptase (1:100; Calbiochem/EMD Millipore), rabbit anti c-Met (1:30; Leica Microsystems Inc.) and rabbit anti-phospho-cMet (1:200; Abcam). As negative controls, non-immune mouse IgG, rabbit IgG or goat IgG were used (Sigma; adjusted to same final concentration as specific primary antibodies). Isolation of primary mammary epithelial cells Tumour tissue was removed aseptically, minced and digested with hyaluronidase (300 U ml −1 ; EMD Chemicals) and collagenase (2 mg ml −1 ; Worthington Biochemical Corporation) added to growth medium containing Ham’s F12:DMEM (Corning Cellgro) supplemented with 5% FCS (Atlanta Biologicals), insulin (10 μg ml −1 ), EGF (10 ng ml −1 ), transferrin (10 μg ml −1 ; Lonza) and hydrocortisone (1 μg ml −1 (Atlanta Biologicals) and incubated for 2 h at 37 °C. Normal primary mammary cells were isolated from inguinal glands 4 and 9 and digested as above for 30 min at 37 °C. Primary epithelial cells or carcinoma cells were then isolated by centrifugation and plated in growth medium [30] , [54] . Growth medium was supplemented with Penicillin/Streptomicin/ Gentamicin (Thermo Scientific). Human breast cancer cell lines The SUM159 and SUM229 cell lines were a gift from Dr Stephen Ethier (Medical University of South Carolina). The HCC1937 and BT20 breast cancer cells were purchased from American Type Culture Collection. SUM159 and SUM229 cells were grown in 5% IH media (Ham’s F-12 media, supplemented with 5% FBS, 1 μg ml −1 hydrocortisone and 5 μg ml −1 insulin), BT-20 cells were grown in Eagles+NEAA media (Eagle’s MEM with 2 mM L-glutamine and Earle’s BSS adjusted to contain 1.5 g l −1 sodium bicarbonate, 0.1 mM non-essential amino acids, 1 mM sodium pyruvate and 10% FBS), SUM190 cells were grown in SFIH media (Ham’s F-12 media, supplemented with 1 μg ml −1 hydrocortisone and 5 μg ml −1 insulin, 5 mM ethanolamine, 10 mM HEPES, 5 μg ml −1 transferrin, 10 nM triodo-thyronine, 50 μM sodium selenite and 5% BSA) and HCC 1937 cells were grown in RPMI+L-GLUT media (RPMI-1640 media with 2 mM L-glutamine adjusted to contain 1.5 g l −1 sodium bicarbonate, 4.5 g l −1 glucose, 10 mM HEPES, 1 mM sodium pyruvate and 10% FBS). Matriptase synthetic inhibitor A selective, slow, tight-binding inhibitor of matriptase containing a ketobenzothiazole serine trap (IN-1) was designed based on the auto-catalytic domain (RQAR) of matriptase. Details on the synthesis and characteristics of the inhibitor have been described previously [46] . Pro-HGF/SF activation assays Pro-HGF/SF was produced in the immortalized human fibroblasts cell line, RMF-HGF [35] , [55] . The cells were maintained in DMEM containing high glucose and supplemented with 10% fetal bovine serum, penicillin/streptomycin and 2 mM L-glutamine (all from Invitrogen Corporation). To collect the pro-HGF/SF, the cells were washed twice with sterile PBS, incubated for 8 h in serum-free DMEM, after which the medium was replaced by fresh serum-free DMEM. The conditioned medium was collected after 72 h, aliquoted and stored at −80 °C. To determine the quality and concentration of each preparation, 40 μl of the conditioned medium was loaded on 4–12% reducing SDS–polyacrylamide gel electrophoresis (SDS–PAGE) and analysed by western blotting using a goat-anti human HGF primary antibody (R&D Systems, 1:1,000) with human recombinant active HGF (R&D Systems) as a loading control. Human breast cancer cell lines or primary mouse MMTV-PymT mammary carcinoma cells were plated in six-well plates and grown to confluence. Cells were then serum starved for a minimum of 3 h. The media were changed to either fresh serum-free media, serum-free media with 100 ng ml −1 recombinant active two-chain HGF/SF (R&D Systems) or pro-HGF/SF with or without either 2 μM Aprotinin (MP Biomedicals, LLC), 20 μM Leupeptin (Fisher Bioreagents), 60 nM HAI-1, 40 nM HAI-2 (R&D Systems) or 1 μM IN-1 (ref. 33 ). Inhibitors were added concomitantly with either pro-HGF/SF or HGF/SF, with the exception of IN-1, where the cells were pre-incubated for 30 min before growth factor stimulation. 3D cell culture Cells were plated on Matrigel Matrix Growth Factor Reduced (BD Biosciences) with serum-free Mammary Epithelial Cell Growth Medium (MEGM; Lonza) containing the BulletKit growth supplement (BPE, hydrocortisone, GA-1000, Insulin). An overlay of MEBM growth media containing 2% Matrigel Matrix Growth Factor Reduced was added 1 h after seeding [56] . Spheroids were allowed to form overnight before addition of 100 ng recombinant HGF/SF (R&D Biosystems) or pro-HGF-conditioned media. After treatment, cells were stained with 5 μM Cell Tracker Orange (Invitrogen) for 45 min and Hoechst 33342 (Life Technologies Carlsbad) for 5 min before imaging. Confocal images were acquired on a Zeiss LSM 780 scope at the Microscopy Imaging and Cytometry Resources Core at the Wayne State University School of Medicine. Light microscopy pictures were acquired using a Nikon TMS microscope courtesy of Dr Hyeong-Reh Kim (Department of Pathology, Wayne State University). RNAi silencing For matriptase knockdown in SUM229, BT20 and HCC1937 breast cancer cells, three independent Stealth RNAi siRNA duplexes (Invitrogen) targeting matriptase (siM1=ST14HSS186125, siM2=ST14HSS186126 siM3=ST14HSS110268) were used [5] . Two independent Stealth RNAi siRNA duplexes targeting uPA (siuPA1=PLAUHSS10878, siuPA2= PLAUHSS10876). Matched %GC negative controls (12935-300 and 12935-400) were used. Cells were transfected using Lipofectamine RNAiMAX (Invitrogen) according to the manufacturer’s instructions. Two days after transfection, the cells were serum starved and used in the pro-HGF/HGF activation assays, in the 3D invasion assays and in the proliferation assays. Transient transfection of SUM159 cells SUM159 cells growing in six-well plates were transfected when they reached 85% confluency using Lipofectamine LTX (Invitrogen) according to the manufacturer’s protocol. The DNA construct used was the mammalian expression vector, pcDNA3.1 containing full-length human matriptase cDNA (a generous gift from Dr Stine Friis, NIH) [57] . Western blot analysis Mouse tissues were snap frozen and homogenized in ice-cold RIPA lysis buffer (150 mM NaCl, 50 mM Tris, 1% NP-40, 0.1% SDS, pH 7.4) with protease inhibitor cocktail (Sigma-Aldrich) and phosphatase inhibitor (Sodium Orthovanadate, Sigma-Aldrich). Cultured mouse and human cells were lysed in ice-cold RIPA buffer with protease inhibitor cocktail and phosphatase inhibitor. Protein concentrations were determined by BCA assay (Pierce) and lysates were separated by 4–12% reducing SDS–PAGE and blotted onto polyvinylidene difluoride membranes (Invitrogen). The following primary antibodies were used for detection: sheep anti-matriptase (1:500; R&D Systems), rabbit anti-matriptase (1:1,000; Calbiochem/EMD Millipore), rabbit anti-phospho cMet (1:500), anti-phospho Gab1 (1:1,000), anti-Gab1 (1:1,000 dilution), anti-phospho Akt (1:1,000), anti-Pan Akt (1:1,000), mouse anti-human cMet (all from Cell Signaling Technology), rabbit anti-uPA (1:500; Abcam) and mouse anti-β-actin (Sigma, 1:1,000). Recombinant human pro-uPA was from American Diagnostica Inc. For detection, secondary antibodies conjugated with either alkaline phosphatase (Sigma) or horseradish peroxidase (Chemicon) in combination with either the chromogenic substrate nitro-blue tetrazolium and 5-bromo-4-chloro-3'-indolyphosphate solutions (Roche; for analysis of human breast cancer cell and primary mammary carcinoma cell extracts) or Super-Signal West Femto Chemiluminescent Substrate (Pierce; for analysis of whole tissue extracts of mammary glands and mammary tumours) were used. Examples of non-cropped scans of western blot membranes are shown in Supplementary Figs 9–11 . Proliferation assays in human breast cancer cell lines A total of 30,000 human breast cancer cells were seeded in a six-well plates and serum starved overnight before stimulation with 100 ng ml −1 active HGF or pro-HGF for 24 h. Thereafter, cells were trypsinized and recounted using a haemocytometer. In the matriptase inhibition assay using IN-1, the synthetic inhibitor was added concomitantly with active HGF or pro-HGF. Matriptase gelatin zymography Serum-free medium conditioned for 4 days by mouse mammary primary cells was collected, centrifuged to remove cell debris and dialysed against distilled water overnight at 4 °C. The dialysed samples were lyophilized, and the dried protein powder was dissolved in a 1/100 volume of the initial conditioned medium in 20 mM Tris-HCl (pH 7.5). Concentrated medium was separated by SDS–PAGE under nonreducing conditions, and the gels (containing 0.1% gelatin) were subsequently incubated in renaturation buffer (50 mM Tris-HCl at pH 7.5, 100 mM NaCl and 2.5% Triton X-100) for 1.5 h followed by 30 min in EDTA buffer (50 mM Tris-HCl at pH 7.5, 0.5 mM EDTA) to eliminate matrix metalloproteinase. The gels were incubated at 37 °C for 16 h in developing buffer (50 mM Tris-HCl at pH 7.5 with 5 mM CaCl 2 ), and stained with Coomassie Brilliant Blue to detect zones of gelatinolysis. Statistical analysis All analyses were performed and graphs generated using Prism 5 software (GraphPad Software Inc.). For comparisons between two groups, Student’s t -test was used. Non-parametric data were compared using the Mann–Whitney test. For correlation data, two estimators of association were used. The tetrachoric correlation coefficient assumes that the variables, matriptase and c-Met, in this case, are normally distributed but that they have been dichotomized. Kendall’s tau does not have the assumption of normality and is a measure of concordance. Both measures have a theoretical range from −1 to 1. How to cite this article: Zoratti, G. L. et al. Targeting matriptase in breast cancer abrogates tumour progression via impairment of stromal-epithelial growth factor signalling. Nat. Commun. 6:6776 doi: 10.1038/ncomms7776 (2015).